Synthetic retinal analogues modify the spectral and kinetic characteristics of microbial rhodopsin optogenetic tools Optogenetic tools have become indispensable in neuroscience to stimulate or inhibit excitable cells by light. Channelrhodopsin-2 (ChR2) variants have been established by mutating the opsin backbone or by mining related algal genomes. As an alternative strategy, we surveyed synthetic retinal analogues combined with microbial rhodopsins for functional and spectral properties, capitalizing on assays in C. elegans , HEK cells and larval Drosophila . Compared with all- trans retinal (ATR), Dimethylamino-retinal (DMAR) shifts the action spectra maxima of ChR2 variants H134R and H134R/T159C from 480 to 520 nm. Moreover, DMAR decelerates the photocycle of ChR2(H134R) and (H134R/T159C), thereby reducing the light intensity required for persistent channel activation. In hyperpolarizing archaerhodopsin-3 and Mac, naphthyl-retinal and thiophene-retinal support activity alike ATR, yet at altered peak wavelengths. Our experiments enable applications of retinal analogues in colour tuning and altering photocycle characteristics of optogenetic tools, thereby increasing the operational light sensitivity of existing cell lines or transgenic animals. Since the initial description of light activation of excitable cells by Channelrhodopsin-2 (ChR2), both in cultured mammalian neurons [1] , [2] , [3] and in vivo in Caenorhabditis elegans ( C. elegans ) [4] , optogenetics has revolutionized research in various biological fields [5] , [6] , [7] , [8] , [9] . Optogenetics combines genetically encoded, light-sensitive proteins and photostimulation for exogenous control of specific cell functions [1] , [2] , [10] in organotypic cultures and intact animals [4] , [11] , [12] . ChR2 has proven highly useful in the study of complex neuronal processes, due to the millisecond precision of triggering neuronal activity [1] , [13] , as well as the need for expression of just a single, small protein. In recent years, various rhodopsin variants have been generated or retrieved from novel algal genome databases [7] , [14] . They can be divided into three main classes: (I) ion pumps (for example, NpHR [12] , [15] , [16] , Mac and Arch3 (refs 17 , 18 )) that pump Cl − inward or H + outward and thereby mediate hyperpolarization; (II) cation channels (for example, ChR2 (refs 12 , 14 , 19 , 20 )) that function as membrane depolarizers; or (III) recently generated ChR2 variants that show Cl − conductance and can counteract depolarization (for example, ChloC [21] and iC1C2 (ref. 22 )). Rhodopsins are conjugates between a seven-transmembrane domain apoprotein, forming an internal, hydrophobic pocket and a photoisomerizable chromophore [23] . In Chlamydomonas reinhardtii , where ChR was originally discovered, all- trans retinal (ATR) is the incorporated pigment [24] , [25] . ATR naturally occurs in mammalian tissue [26] , [27] or can easily be supplied to animals that do not have sufficient retinal (for example, C. elegans , larval Drosophila ). The ability of rhodopsins to be activated by light is based on the characteristic absorption spectrum of their chromophore, which depends on the molecular environment of ATR inside the protein. When ATR (embedded in a microbial rhodopsin) absorbs a photon, it isomerizes to 13- cis retinal, which causes a conformational change and gating of the opsin [28] . A recent focus of opsin research has been to shift its action spectrum, either to long-wavelength absorption [19] , [29] , [30] , [31] , [32] , [33] or to wavelengths below its maximum of 470 nm (refs 33 , 34 ). This will facilitate the independent activation of different cell types or allow to combine photoactivation with the imaging of neuronal activity using genetically encoded Ca 2+ indicators (GECIs) [35] , [36] , [37] , [38] . Currently used GECIs, based on GFP (green fluorescent protein), are often excited at the same wavelength as ChR2, apart from RCaMP [38] or R-GECO [39] , which are based on red fluorescent mRuby or mApple, respectively. Yet, R-GECO shows photoswitching properties upon blue-light illumination, which complicates its use in combination with ChR2. For spectral separation, it would be desirable to shift the absorption of ChR to a wavelength outside the GECI excitation range. However, reaching this aim is complicated by the broad spectra of the α-band and the blue-shifted smaller β-band. Thus far, this could not be altered by mutating the protein backbone. An absorption shift is also of interest for independent control in the same animal, using a second rhodopsin. Last, shifting the absorption to higher wavelengths facilitates the penetration depth of the stimulating light in large animals, as it reduces scattering in the tissue and absorption by haemoglobin. Strategies to achieve a spectral shift or otherwise modified properties include varying the retinal-binding pocket of the apoprotein by single or multiple point mutations [5] , [7] , [10] , [13] , [14] , [15] , [19] , [32] (for example, ChR2(T159C) (ref. 40 )), generating chimeras of different ChRs (for example, C1V1 (refs 14 , 20 )), or screening algal genomes for novel ChRs [33] . These variants have diverse characteristics and may, in addition to or instead of colour tuning, feature an extended lifetime of the open-state (ChR2(C128S) (refs 41 , 42 )) or high expression levels and high-efficiency kinetics (ChR2(H134R/T159C) (refs 14 , 20 )). However, colour tuning is often accompanied by unwanted side effects, such as decreased current amplitude [43] or decelerated kinetics [19] . An alternative option to shift the absorption spectrum or generate kinetic changes is to modify the chromophore by supplementing the medium or animal diet with retinal analogues. Synthetic retinal analogues can be generated by altering the length of the π -electron system or the structure of the polyene ‘backbone’ of the molecule; some of these have been tested for ChR activity in living algae [24] , [25] , [29] , [44] . Reconstitution of Arch3 and four ChR variants with A2 retinal, which carries an extra double bond, resulted in functional pigments with enhanced long-wavelength sensitivity [29] . Extensive work on bacteriorhodopsin (BR) [45] , [46] , [47] , [48] , [49] using synthetic retinal analogues suggests that many other retinal analogues, particularly those with ring modifications, might be applicable for the purpose of chromophore substitution. However, in most cases, it was only shown that the absorption maximum was shifted, without analysing the rhodopsin function. Due to its transparency, C. elegans is particularly well suited for optogenetic analyses, and chromophore replacement is easily achieved as ATR has to be provided as a supplement in the diet [4] . Here we tested eight synthetic retinal analogues for their ability to reconstitute the function of selected optogenetic tools, including de- and hyperpolarizers. We analysed whether the analogues would allow shifting the excitation wavelength or the extent of light-induced effects. In ChR2(H134R) (ref. 50 ), the retinal analogue Dimethylamino-retinal (DMAR) can reconstitute a fully functional actuator and it expands its spectral sensitivity to longer wavelengths. Due to the broad action spectrum, ChR2-DMAR will likely not enable pairing with GECIs without optical crosstalk, unless these are very blue-shifted. Behavioural and electrophysiological analysis of body wall muscles (BWMs) in C. elegans show significantly prolonged kinetics, leading to an overall increase in charge transfer. Similar results were found during electrophysiological studies on HEK cells. In other ChR variants, such as ChR2(H134R/T159C), DMAR slows down the photocycle even more, causing increased operational light sensitivity of the cells, whereas it does not support function in the spectrally red-shifted C1V1. DMAR also enhances ChR2 function in larval Drosophila , confirming that it can be used in additional model systems. In combination with the hyperpolarizers Arch3 and Mac, naphthyl-retinal and thiophene-retinal show effects on C. elegans behaviour and on current amplitudes in HEK cells that are comparable or even superior to ATR, with naphthyl-retinal for example causing a significant blue shift in Arch3. In summary, the use of retinal analogues is a complementary strategy to obtain rhodopsin-based optogenetic tools with modified characteristics, particularly in already existing cell or animal lines. Synthetic retinal analogues affect the peak absorption of ChR2 From a range of artificial retinal analogues that had been investigated previously, we chose seven that caused a shift in the absorption maxima of BR or ChR2 compared with ATR (analogues II–VII (refs 47 , 51 , 52 ); analogue IX: trimethoxy-retinal [53] ). An additional analogue (VIII: thiophene-retinal) was newly synthesized from a previously known precursor [54] ( Fig. 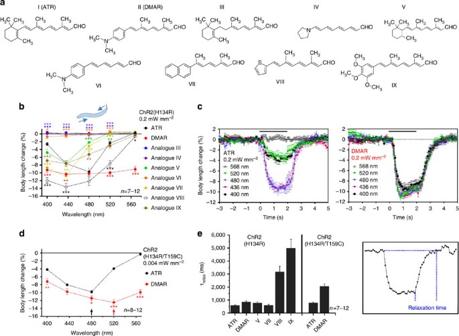Figure 1: ATR variants analysed in combination with ChR2 inC. elegansmuscle. (a) Chemical structures of ATR and retinal analogues tested in this study. (b) Action spectra of photostimulated body length changes (contractions; see inset) in animals expressing ChR2(H134R) in BWMs. The animals were provided with 250 μM ATR (black;n=7 (400/480 nm) or 8 (436/520/568 nm)) or retinal analogue II (n=10), III (n=10), IV (n=10), V (n=12), VI (n=10), VII (n=12), VIII (n=8 (480/568 nm) or 9 (400/436/520 nm)) or IX (n=7 (400 nm), 8 (480/520 nm) or 9 (436/568 nm)). Body length was analysed at five wavelengths (400, 436, 480, 520 and 568 nm; 0.2 mW mm−2) and changes were measured relative to the initial length of unstimulated animals. Statistically significant differences are relative to ATR at the respective wavelength. (c) Time course of body length changes for animals raised in the presence of ATR (left) and DMAR (right). The black bar marks the period of illumination (n=7). (d) Action spectra of photostimulated body length changes in animals expressing ChR2(H134R/T159C) in BWMs. The animals were provided with ATR (black;n=8 (520 nm), 9 (400/436 nm), 10 (480 nm) or 12 (568 nm)) or DMAR (red;n=12). Body length was analysed at five wavelengths (400, 436, 480, 520 and 568 nm) and at reduced light intensity (0.004 mW mm−2). Changes were measured relative to the initial length of unstimulated animals. Statistically significant differences are relative to ATR at the respective wavelength. (e)τrelaxvalues (see inset) of light-stimulated body length changes. Details as inb,d. Time constants were obtained by non-linear fitting for monoexponential decay of body length. Displayed are means±s.e.m. Allnvalues refer to animals. Statistically significant differences are indicated (*P<0.05, **P<0.01, ***P<0.001; one-way analysis of variance (b); Student’st-test (d)). 1a ; Supplementary Table 1 ; Supplementary Methods ). The functionality of these synthetic analogues was analysed in vivo in BWMs of C. elegans expressing the channelrhodopsin variant ChR2(H134R), which has a nearly twofold higher Na + conductance, a twofold lower degree of inactivation and improved expression in C. elegans , resulting in larger photocurrent amplitudes [4] , [55] , [56] . The potential of the retinal analogues was evaluated by measuring changes in the body length due to depolarization-induced contraction of the body following illumination (2 s; 400–568 nm; 0.2 mW mm − 2 ; see Supplementary Fig. 1a for a titration of ATR concentration required for maximal behavioural effects). In the absence of any chromophore ( Supplementary Fig. 1b ) or in nontransgenic animals (no ChR2(H134R) expression) supplemented with retinoids ( Supplementary Fig. 1c ), photostimulation did not cause any significant effects. In contrast, the presence of ATR (250 μM; for details see Methods) and ChR2(H134R) resulted in significant body contractions. The action spectrum featured a maximum at about 480 nm with a 9.7±1.0% ( n =7) reduction in body length ( Fig. 1b ). Some of the synthetic analogues facilitated body contractions similar to ATR (retinal analogues II (DMAR), VII), whereas others evoked weaker effects (V, IX) or even no significant body contractions at all (III, IV, VI). Of all chromophores tested, analogue VIII (thiophene-retinal) enabled the strongest effect (−13.6±0.9% ( n =9); 436 nm), hinting at increased photocurrents and/or extended open-state lifetime ( Fig. 1b ; Supplementary Fig. 2f ). In addition, analogues V, VII, VIII and IX caused a slight shift of the action spectrum maximum to shorter wavelengths compared with ATR (more pronounced function at 436 nm than at 480 nm). Figure 1: ATR variants analysed in combination with ChR2 in C. elegans muscle. ( a ) Chemical structures of ATR and retinal analogues tested in this study. ( b ) Action spectra of photostimulated body length changes (contractions; see inset) in animals expressing ChR2(H134R) in BWMs. The animals were provided with 250 μM ATR (black; n =7 (400/480 nm) or 8 (436/520/568 nm)) or retinal analogue II ( n =10), III ( n =10), IV ( n =10), V ( n =12), VI ( n =10), VII ( n =12), VIII ( n =8 (480/568 nm) or 9 (400/436/520 nm)) or IX ( n =7 (400 nm), 8 (480/520 nm) or 9 (436/568 nm)). Body length was analysed at five wavelengths (400, 436, 480, 520 and 568 nm; 0.2 mW mm − 2 ) and changes were measured relative to the initial length of unstimulated animals. Statistically significant differences are relative to ATR at the respective wavelength. ( c ) Time course of body length changes for animals raised in the presence of ATR (left) and DMAR (right). The black bar marks the period of illumination ( n =7). ( d ) Action spectra of photostimulated body length changes in animals expressing ChR2(H134R/T159C) in BWMs. The animals were provided with ATR (black; n =8 (520 nm), 9 (400/436 nm), 10 (480 nm) or 12 (568 nm)) or DMAR (red; n =12). Body length was analysed at five wavelengths (400, 436, 480, 520 and 568 nm) and at reduced light intensity (0.004 mW mm −2 ). Changes were measured relative to the initial length of unstimulated animals. Statistically significant differences are relative to ATR at the respective wavelength. ( e ) τ relax values (see inset) of light-stimulated body length changes. Details as in b , d . Time constants were obtained by non-linear fitting for monoexponential decay of body length. Displayed are means±s.e.m. All n values refer to animals. Statistically significant differences are indicated (* P <0.05, ** P <0.01, *** P <0.001; one-way analysis of variance ( b ); Student’s t -test ( d )). Full size image DMAR red-shifts the action spectra of ChR2 variants In solution, free DMAR (II) showed a 67-nm bathochromic shift of the peak absorption (449 versus 382 nm; Supplementary Fig. 3 ) and seemed to be most promising for application in animals. When incorporated into ChR2(H134R), it mediated light-evoked body contractions in C. elegans at 480 nm, similar to those evoked by ATR (−10.2±0.4%; n =10; Fig. 1b,c ). However, the action spectrum was broader and red-shifted. On further reduction of the light intensity from 0.2 to 0.015 mW mm − 2 , DMAR still supported strong contractions both at 480 and at 520 nm (−11.6±0.4%; n =12; Supplementary Fig. 2a,b ), indicating a >20-nm red-shifted peak activity and overall improved operational sensitivity of the muscle cell ( Supplementary Fig. 2c ; see below). Furthermore, DMAR showed excellent photostability during multiple cycles of illumination ( Supplementary Fig. 4 ). A highly efficient variant of ChR2 is (H134R/T159C), which combines two mutations leading to increased photocurrents [1] , [20] . Previously, we have shown that C. elegans expressing this rhodopsin in BWMs exhibit stronger body contractions than those expressing ChR2(H134R) at all wavelengths tested (400–520 nm) (ref. 20 ). Therefore, it is possible to photostimulate cells at very low light intensities. At 0.004 mW mm −2 , ChR2(H134R/T159C) mediated strong contractions with the ATR chromophore, again reaching a maximum at 480 nm (−9.8±0.4%; n =10; Fig. 1d ; Supplementary Fig. 5 ), whereas at 520 nm contractions were considerably smaller (−3.9±0.1%; n =8). However, when animals were supplemented with DMAR, it still enabled strong depolarization above 560 nm (−9.9±0.6%; 568 nm; n =12). Thus, ChR2(H134R/T159C) could be efficiently activated even at 568 nm at low light intensity when using DMAR instead of ATR. Furthermore, for both of these ChR2 variants, we observed slowed kinetics of body relaxation following the end of the light stimulus, if ATR was replaced by DMAR ( Fig. 1e ). In animals expressing ChR2(H134R), the τ relax value increased from 580±50 ms (ATR; n =7; 480 nm) to 850±80 ms (DMAR; n =10; 520 nm). The same tendency was observed in animals expressing ChR2(H134R/T159C), where τ relax increased from 780±50 ms (ATR; n =10; 480 nm) to 2,052±180 ms (DMAR; n =7; 520 nm). The slowing down of body relaxation hints at a slower closing of ChR2, which causes prolonged muscle contraction. This slightly delays acute relaxation following the light stimulus, but in a way that does not compromise the behavioural analysis. The single-mutant ChR2(T159C) was shown to be highly efficient in Xenopus oocytes [40] ; however, in C. elegans it was shown to be much less efficient [20] and we could not improve this using DMAR instead of ATR (−6.3±0.9%; 480 nm; n =10; Supplementary Fig. 6a,b ). C1V1(E122T/E162T), a chimera from ChR1s of C. reinhardtii and V. carteri [14] , reliably permits photodepolarization at red-shifted excitation between 520 and 580 nm, when supplemented with ATR [20] . However, surprisingly, the C1V1–DMAR combination was non-functional and did not promote body contractions in light (−0.6±0.6%; 480 nm; n =6; Supplementary Fig. 6c,d ). Thus, specific retinal analogues may function in one, but not another, rhodopsin, possibly enabling orthogonal combinations in animals. DMAR slows down channel kinetics To further characterize the extent and kinetics of photocurrents in DMAR-supplemented animals expressing ChR2(H134R) and ChR2(H134R/T159C), we performed whole-cell patch-clamp studies in C. elegans BWMs. At 470 nm, the transient peak current in animals supplemented with DMAR reached 120±22 pA ( n =7; Fig. 2a,c ), while in animals cultivated with ATR, peak currents reached 155±22 pA ( n =7). However, due to slower kinetics, the overall charge transfer was higher with DMAR ( Fig. 2d ). In contrast, at 525 nm, peak currents after photoactivation were significantly smaller for ATR (86±13 pA; n =7) versus DMAR supplementation (142±28 pA; n =8) and, furthermore, charge transfer at 525 nm was larger for DMAR (−126.0±29.2 pC; n =8) than for ATR (−72.8±10.7 pC; n =7). These electrophysiological differences most likely correspond to the increased efficiency of ChR2(H134R) supplemented with DMAR at wavelengths >470 nm, as discovered in behavioural assays ( Fig. 1b ), as well as to the observed increase in operational light sensitivity of the BWMs ( Supplementary Fig. 2a,b ). 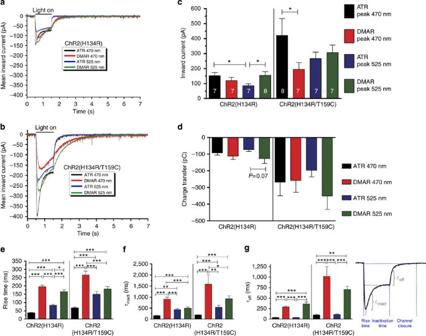Figure 2: Electrophysiological analysis of photocurrents inC. elegansBWMs. All animals were grown either on 250 μM ATR or DMAR. Cells were photoactivated by a 1-s light pulse (0.2 mW mm−2) at 470 or 525 nm, and currents recorded at a holding potential of −60 mV. (a) Mean inward currents following light stimulation in animals expressing ChR2(H134R) in BWMs. During photoactivation, the peak current decays to a lower steady state level. (b) Mean inward currents following light stimulation in animals expressing ChR2(H134R/T159C) in BWMs. (c) Mean peak currents of animals expressing either ChR2(H134R) (left) or ChR2(H134R/T159C) (right) in BWMs. Numbers in the bars indicatenvalues for each experiment. (d) Charge transfer at 525 nm was increased in animals grown on DMAR. (e) The rise time (time to reach peak after onset of light stimulus; see inset on the right) featured significantly increased values for animals grown on DMAR. (f) Comparison of time constants for inactivation during continuous illumination (τinact). (g) Channel closure after the end of photostimulation featured significantly prolongedτoffvalues in animals grown on DMAR. Time constants were obtained by non-linear fitting for monoexponential decay of inward current changes. Displayed are means±s.e.m. (nvalues as indicated inc). Allnvalues refer to cells. Statistically significant differences are indicated (*P<0.05, **P<0.005, ***P<0.001; one-way analysis of variance). Figure 2: Electrophysiological analysis of photocurrents in C. elegans BWMs. All animals were grown either on 250 μM ATR or DMAR. Cells were photoactivated by a 1-s light pulse (0.2 mW mm −2 ) at 470 or 525 nm, and currents recorded at a holding potential of −60 mV. ( a ) Mean inward currents following light stimulation in animals expressing ChR2(H134R) in BWMs. During photoactivation, the peak current decays to a lower steady state level. ( b ) Mean inward currents following light stimulation in animals expressing ChR2(H134R/T159C) in BWMs. ( c ) Mean peak currents of animals expressing either ChR2(H134R) (left) or ChR2(H134R/T159C) (right) in BWMs. Numbers in the bars indicate n values for each experiment. ( d ) Charge transfer at 525 nm was increased in animals grown on DMAR. ( e ) The rise time (time to reach peak after onset of light stimulus; see inset on the right) featured significantly increased values for animals grown on DMAR. ( f ) Comparison of time constants for inactivation during continuous illumination ( τ inact ). ( g ) Channel closure after the end of photostimulation featured significantly prolonged τ off values in animals grown on DMAR. Time constants were obtained by non-linear fitting for monoexponential decay of inward current changes. Displayed are means±s.e.m. ( n values as indicated in c ). All n values refer to cells. Statistically significant differences are indicated (* P <0.05, ** P <0.005, *** P <0.001; one-way analysis of variance). Full size image In comparison, the ChR2(H134R/T159C)/ATR combination generally caused much stronger photocurrents (470 nm; ATR: 421±112 pA; n =8; DMAR: 195±46 pA; n =7; Fig. 2b,c ). Other effects of replacing ATR with DMAR were similar to those observed for ChR2(H134R). At 470 nm, overall charge transfer was similar for both retinals (ATR: −268±82 pC; n =8; DMAR: −258±71 pC; n =7; Fig. 2d ). However, when switching to higher wavelength, the overall charge transfer was increased by 78% with DMAR (ATR: −196±40 pC; n =7; DMAR: −350±81 pC; n =7; 525 nm). In both ChR2 variants, DMAR led to a slowdown in channel kinetics with increased rise time (=time to peak; Fig. 2e ) and τ inactivation values (time constant of current decreasing from peak to steady state; Fig. 2f ). Channel closure decelerated with τ off values increasing from 41±3 ms (ATR; n =7) to 293±22 ms (DMAR; n =7) in animals expressing ChR2(H134R) and from 112±16 ms (ATR; n =7) to 708±74 ms (DMAR; n =7) in animals expressing ChR2(H134R/T159C) ( Fig. 2g ). In particular, because the closing of the channel is influenced to a large extent, a larger proportion of the channels accumulate ChR in the open state ( Supplementary Fig. 2a,b ), causing higher photosensitivity of DMAR-supplemented cells, as previously reported for step function rhodopsins [14] , [41] , [42] , [57] . Testing other retinal analogues Besides DMAR, the retinal analogues V and VII (naphthyl-retinal) mediated maximal body contractions with ChR2(H134R), comparable to those achieved with ATR ( Fig. 1b ). They also slightly slowed down time courses of body relaxation after the light was turned off, increasing τ relax values from 520±110 ms (ATR; n =10) to 770±80 ms ( n =12) and 590±78 ms ( n =12), respectively ( Fig. 1e ). An even stronger deceleration was obtained for thiophene-retinal (VIII; which also enabled the strongest contractions) and for trimethoxy-retinal (IX), featuring τ relax values of 3,163±440 ms ( n =8) and 4,980±700 ms ( n =7). For all these four retinal analogues, based on behavioural assays, the action spectra peaks featured a hypsochromic shift from 480 nm (ATR) toward 436 nm. When combining retinal analogues V and VII with the highly efficient ChR2(H134R/T159C), contractions of −11.6±1.2% ( n =10; Supplementary Fig. 7a,d ) and −14.2±0.5% ( n =10; Supplementary Fig. 8a,d ) were achieved, respectively. In contrast, combination with ChR2(T159C) elicited only reduced contractions (−3.9±0.8%; n =10; Supplementary Fig. 7c ; −8.3±0.5%; n =10; Supplementary Fig. 8c , respectively). Because ChR2(T159C) also reached only low effectiveness in combination with ATR and DMAR as discussed above ( Supplementary Fig. 6a,b ), our results suggest that this rhodopsin generally has only low efficiency in C. elegans , at least with the retinal analogues tested. Absorption shifts and kinetic changes in HEK cells Retinal analogues can also be used in other systems to alter rhodopsin properties. This should be readily achievable when there is little or no endogenous retinal, as in Drosophila (see below). However, mammalian cells may also benefit from retinal analogues to modify rhodopsin properties for specific applications. Thus, we attempted to reduce endogenous ATR levels in cultured HEK-293 cells by the removal of retinoid sources from the culture media, and instead added retinal analogues. We then assessed the functionality of wild-type ChR2 (as the H134R variant does not express well in HEK cells) by recording photocurrents and compared the electrophysiological parameters to those observed in C. elegans , using the most promising retinal analogues. Current–voltage relationships of patch-clamped HEK cells stably expressing ChR2 were recorded at holding potentials ranging from −60 to +40 mV during illumination (300 ms; 465 nm; 0.119 mW mm −2 ). Even without the addition of retinal, photostimulation led to small currents at −60 mV (−291±88 pA; n =6; Fig. 3f ), suggesting that our attempted reduction of endogenous ATR was incomplete. ChR currents without added retinal, but supplemented with 10% fetal bovine serum, have been previously reported in HEK cells [58] . However, supplementation with ATR (1 μM; Fig. 3a ) led to strongly increased peak currents of −1,674±271 pA ( n =7). HEK cells that had been exposed to DMAR (1 μM; Fig. 3b ), naphthyl-retinal (analogue VII; Fig. 3c ) or thiophene-retinal (analogue VIII; Fig. 3d ) exhibited reduced currents compared with those exposed to ATR. This was most evident for DMAR, where current amplitudes showed a significant decrease to −437±81 pA ( n =6; Fig. 3f ). 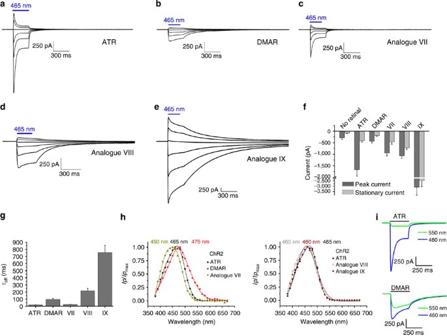Figure 3: Electrophysiological analysis of ChR2 photocurrents in HEK cells. Current–voltage relationships of patch-clamped HEK cells grown in the presence of 1 μM ATR (a), DMAR (b), retinal analogue VII (c), VIII (d) or IX (e) were recorded at different holding voltages (−60, −40, −20, 0, +20 and +40 mV). Cells were illuminated at 465 nm for 300 ms (0.150 mW mm−2). The original traces are displayed. (f) Comparison of absolute current amplitudes at 465 nm (0.150 mW mm−2; holding potential −60 mV) in the absence of any retinal (n=6) or in the presence of ATR (n=7), DMAR (n=6), analogue VII (n=4), analogue VIII (n=7) and analogue IX (n=5). The mean peak currents (dark grey) and stationary currents (light grey) are displayed. (g)τoffvalues at 465 nm (0.150 mW mm−2; holding potential −60 mV). (h) Action spectra of peak photocurrents between 380 and 670 nm (with additional 10% grey filter, equal photon flux of 2.81 × 1013photons s−1mm−2, holding potential −60 mV) for ATR (n=7), DMAR (n=7), analogue VII (n=6), analogue VIII (n=4) or analogue IX (n=6). Displayed are means±s.e.m. (i) Comparison of currents (holding potential −60 mV) in the presence of either ATR (1 μM) or DMAR at 460 and 550 nm. At 460 nm (0.158 mW mm−2), currents in the presence of ATR were significantly larger, while at 550 nm (0.132 mW mm−2), currents in the presence of DMAR were significantly larger. The original traces are displayed. Allnvalues refer to cells. Figure 3: Electrophysiological analysis of ChR2 photocurrents in HEK cells. Current–voltage relationships of patch-clamped HEK cells grown in the presence of 1 μM ATR ( a ), DMAR ( b ), retinal analogue VII ( c ), VIII ( d ) or IX ( e ) were recorded at different holding voltages (−60, −40, −20, 0, +20 and +40 mV). Cells were illuminated at 465 nm for 300 ms (0.150 mW mm −2 ). The original traces are displayed. ( f ) Comparison of absolute current amplitudes at 465 nm (0.150 mW mm −2 ; holding potential −60 mV) in the absence of any retinal ( n =6) or in the presence of ATR ( n =7), DMAR ( n =6), analogue VII ( n =4), analogue VIII ( n =7) and analogue IX ( n =5). The mean peak currents (dark grey) and stationary currents (light grey) are displayed. ( g ) τ off values at 465 nm (0.150 mW mm −2 ; holding potential −60 mV). ( h ) Action spectra of peak photocurrents between 380 and 670 nm (with additional 10% grey filter, equal photon flux of 2.81 × 10 13 photons s −1 mm −2 , holding potential −60 mV) for ATR ( n =7), DMAR ( n =7), analogue VII ( n =6), analogue VIII ( n =4) or analogue IX ( n =6). Displayed are means±s.e.m. ( i ) Comparison of currents (holding potential −60 mV) in the presence of either ATR (1 μM) or DMAR at 460 and 550 nm. At 460 nm (0.158 mW mm −2 ), currents in the presence of ATR were significantly larger, while at 550 nm (0.132 mW mm −2 ), currents in the presence of DMAR were significantly larger. The original traces are displayed. All n values refer to cells. Full size image How this compares with the superior effects of DMAR in C. elegans is currently unclear. The differences may be imposed by using wild-type ChR2 versus ChR2(H134R), the size of the cells (HEK cells ~15–30 μm; BWMs ~100 × 15 μm) and also the different ionic compositions of the solutions used. Chromophore access to the protein may furthermore depend on host-specific factors or, though less likely, retinal analogues could be modified in a host-specific manner. Other retinal analogues also had different relative effectiveness in HEK cells compared with C. elegans : naphthyl-retinal (VII) and thiophene-retinal (VIII) supported ChR2 peak currents of −948±123 pA ( n =4) and −1,066±120 pA ( n =7), respectively ( Fig. 3f ). Yet the strongest photocurrents (nearly twice as large as ATR-dependent currents) were induced by trimethoxy-retinal (analogue IX; −3,068±768 pA; n =5; Fig. 3e,f ), which was not one of the most effective retinals in C. elegans ( Fig. 1b ). While stationary currents reached only 25% of the peak currents in the presence of ATR, they reached 44% in the presence of DMAR and even 80% with trimethoxy-retinal. These characteristics were related to slow photocycle kinetics with significantly increased closing times ( Fig. 3g ); this was in good agreement with results from C. elegans ( Fig. 1e , Fig. 2g ). In HEK cells, the τ off measured for ATR was 18±2 ms ( n =8); this was increased to 26±2 (naphthyl-retinal; n =3), 97±12 (DMAR; n =6), 217±35 (thiophene-retinal; n =8) and even 753±102 ms (trimethoxy-retinal; n =6). Precisely resolved action spectra of the retinal analogues in HEK cells were determined by measuring photocurrents at different wavelengths (380–670 nm; holding potential −60 mV; Fig. 3h ). The DMAR action spectrum was broader and slightly shifted to longer wavelengths (maximum 475 nm) compared with ATR (maximum 465 nm). Thus, DMAR’s shift in the action spectrum was much smaller than the shift of the absorption of free DMAR compared to ATR ( Supplementary Fig. 3 ). Nevertheless, photocurrents at 460 nm were larger for cells grown on ATR, while photocurrents at 550 nm were larger for cells grown on DMAR ( Fig. 3i ). In contrast, the action spectra of cells cultivated with naphthyl-retinal (VII), thiophene-retinal (VIII) and trimethoxy-retinal (IX) were slightly blue-shifted, with maxima at 450, 460 and 460 nm, respectively ( Fig. 3h ). These results corresponded well to the C. elegans behavioural data ( Fig. 1b ). DMAR causes a red-shift of excitation in larval Drosophila Optogenetic neuronal depolarization using rhodopsins is a readily functional technique in larval Drosophila [8] , [59] , [60] . Here we expressed ChR2(H134R) (ref. 59 ) ubiquitously under control of an actin promoter using the Gal4–UAS system [61] . Larvae raised on medium containing 125 μM ATR ( n ≥5) showed strong body contractions during illumination, entirely immobilizing the larvae, with a peak of efficiency at 465–525 nm at an irradiance of 0.02 mW mm − 2 ( Fig. 4 ). Larvae raised on 125 μM DMAR ( n =10) featured similar behaviour, but strong contractions were achieved even at 0.01 mW mm − 2 ( P =0.013). Though a high percentage of ATR-fed larvae ( n ≥6) showed clear contractions at this intensity, in contrast to DMAR-fed larvae the observed contractions were much weaker. No reliable contractions were observed in the absence of retinoids (control with diluent EtOH; n ≥8) or for parental control strains carrying either ChR2(H134R) construct only (UAS:ChR2(H134R)) or Gal4 construct only (Actin-Gal4; 0.1 mW mm − 2 ; DMAR, n ≥7; ATR, n ≥7). On long-wavelength stimulation (590 and 625 nm), a higher percentage of DMAR-fed larvae still featured contractions at strong light intensities (0.1 mW mm − 2 ; P =0.011; n ≥9), whereas only about 30% of ATR-fed larvae contracted strongly ( n ≥7). DMAR mediated strong body contractions even at 625-nm illumination at lower irradiations where ATR was much less effective and only led to strong contraction at the highest intensity used. This demonstrates that, in this key model organism, DMAR induces a red-shift in the efficient absorption wavelength of ChR2 and mediates enhanced sensitivity. 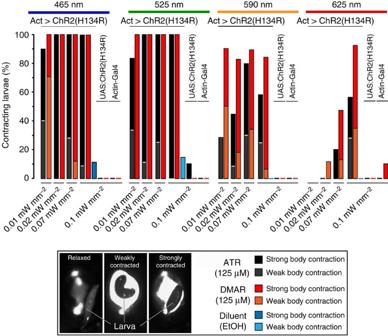Figure 4: Dependency on wavelength and light intensity inDrosophilalarvae. Larvae expressing ChR2(H134R) ubiquitously (Actin-Gal4>UAS:ChR2(H134R)) showed reliable light-induced contractions at 465 and 525 nm at an irradiance of 0.02 mW mm−2when ATR (125 μM) was supplied in the diet (n≥5). At a wavelength of 525 nm, larvae fed with DMAR (125 μM) contracted reliably even at 0.01 mW mm−2(n=10), whereas ATR-fed larvae showed reliable contractions at a light intensity of 0.02 mW mm−2(P=0.013,χ2-test). At longer spectral wavelengths (590 and 625 nm), more than 60% of DMAR-fed larvae (n≥14) still showed contractions at strong light intensities (0.1 mW mm−2), whereas only about 30% of ATR-fed larvae (n≥7) contracted at these wavelengths. No reliable contraction could be observed when only the diluent (EtOH) was supplied to the food (n≥8). Control strains carrying either the UAS:ChR2(H134R) construct only or the Actin-Gal4 construct only did not show contractions, with either DMAR or ATR (n≥7). Body contractions were classified as ‘weakly contracted’ when animals showed clear contractions, but were still able to move, and ‘strongly contracted’ when animals were completely immobilized during the first seconds of irradiation. Allnvalues refer to animals. Figure 4: Dependency on wavelength and light intensity in Drosophila larvae. Larvae expressing ChR2(H134R) ubiquitously (Actin-Gal4>UAS:ChR2(H134R)) showed reliable light-induced contractions at 465 and 525 nm at an irradiance of 0.02 mW mm − 2 when ATR (125 μM) was supplied in the diet ( n ≥5). At a wavelength of 525 nm, larvae fed with DMAR (125 μM) contracted reliably even at 0.01 mW mm − 2 ( n =10), whereas ATR-fed larvae showed reliable contractions at a light intensity of 0.02 mW mm − 2 ( P =0.013, χ 2 -test). At longer spectral wavelengths (590 and 625 nm), more than 60% of DMAR-fed larvae ( n ≥14) still showed contractions at strong light intensities (0.1 mW mm − 2 ), whereas only about 30% of ATR-fed larvae ( n ≥7) contracted at these wavelengths. No reliable contraction could be observed when only the diluent (EtOH) was supplied to the food ( n ≥8). Control strains carrying either the UAS:ChR2(H134R) construct only or the Actin-Gal4 construct only did not show contractions, with either DMAR or ATR ( n ≥7). Body contractions were classified as ‘weakly contracted’ when animals showed clear contractions, but were still able to move, and ‘strongly contracted’ when animals were completely immobilized during the first seconds of irradiation. All n values refer to animals. Full size image Testing Arch3 and Mac in C. elegans and HEK cells A wealth of previous work has shown that retinal analogues modify the properties of rhodopsin proton pumps, particularly BR [62] . Arch3 or Mac are better expressed in eukaryotes and commonly used to hyperpolarize and inhibit excitable cells [12] , [18] . We expressed Arch3 in C. elegans BWMs and recorded effects of photostimulation on body length between 400 and 600 nm (0.2 mW mm −2 ). Hyperpolarization induced body elongation, as muscles became inhibited and relaxed due to the internal hydrostatic pressure of the C. elegans body. Although no photostimulation effects could be observed in the absence of retinal ( Supplementary Fig. 9 ), the presence of ATR mediated a maximal increase in body length during illumination at 568 nm (4.5±0.5%; n =5; Fig. 5a ). The relaxation was maintained during the entire light pulse and returned to the basal level after about 0.5–1 s in the dark ( Supplementary Fig. 9a ). Most analogues were less efficient than ATR with the exception of thiophene-retinal (VIII) that caused increased sensitivity between 400 and 480 nm. 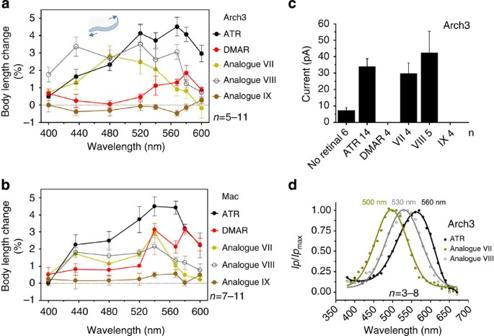Figure 5: Effects onC. elegansBWMs and HEK cells expressing Arch3 and Mac. C. elegansor HEK cells were cultivated in the presence of ATR or various retinal analogues. The chromophores were provided at 100 μM (C. elegans) or 1 μM (HEK cells). (a) Action spectra of body length changes (elongations; see inset) inC. elegansexpressing Arch3 in BWMs. The 2-s illumination was carried out at 400, 436, 480, 520, 540 568, 580 and 600 nm (0.2 mW mm−2). Body length changes were measured relative to the initial length of unstimulated animals. Displayed are means±s.e.m. for ATR (n=5), DMAR (n=5), analogue VII (n=11), analogue VIII (n=9) or analogue IX (n=7). (b) Action spectra of body length changes inC. elegansexpressing Mac in BWMs. Illumination and body length measurements were carried out as for Arch3 (a). Displayed are means±s.e.m. for ATR (n=7), DMAR (n=10), analogue VII (n=11), analogue VIII (n=7) or analogue IX (n=7). (c) Comparison of absolute peak current amplitudes in HEK cells at a holding potential of 0 mV and at the respective action spectra maxima for ATR (565 nm,n=14), DMAR (no signal in action spectra,n=4), analogue VII (500 nm,n=4), analogue VIII (530 nm,n=5), analogue IX (no signal in action spectra,n=4) and in the absence of retinal (565 nm,n=6). Amplitudes of Arch3 were recorded at the highest transmission of 0.080–0.110 mW mm−2(at maximal transmission between 500 and 565 nm). Displayed are means±s.e.m. (d) Action spectra of HEK cells transfected with Arch3-EGFP in presence of ATR (n=3), analogue VII (n=7) or analogue VIII (n=8). DMAR and analogue IX were also tested but did not enable photocurrents. Displayed are stationary currents following photostimulation at a holding potential of 0 mV (equal photon flux for each wavelength of 2.81 × 1014photons s−1mm−2). In (a) and (b)nvalues refer to animals, in (c) and (d)nvalues refer to cells. Figure 5: Effects on C. elegans BWMs and HEK cells expressing Arch3 and Mac. C. elegans or HEK cells were cultivated in the presence of ATR or various retinal analogues. The chromophores were provided at 100 μM ( C. elegans ) or 1 μM (HEK cells). ( a ) Action spectra of body length changes (elongations; see inset) in C. elegans expressing Arch3 in BWMs. The 2-s illumination was carried out at 400, 436, 480, 520, 540 568, 580 and 600 nm (0.2 mW mm −2 ). Body length changes were measured relative to the initial length of unstimulated animals. Displayed are means±s.e.m. for ATR ( n =5), DMAR ( n =5), analogue VII ( n =11), analogue VIII ( n =9) or analogue IX ( n =7). ( b ) Action spectra of body length changes in C. elegans expressing Mac in BWMs. Illumination and body length measurements were carried out as for Arch3 ( a ). Displayed are means±s.e.m. for ATR ( n =7), DMAR ( n =10), analogue VII ( n =11), analogue VIII ( n =7) or analogue IX ( n =7). ( c ) Comparison of absolute peak current amplitudes in HEK cells at a holding potential of 0 mV and at the respective action spectra maxima for ATR (565 nm, n =14), DMAR (no signal in action spectra, n =4), analogue VII (500 nm, n =4), analogue VIII (530 nm, n =5), analogue IX (no signal in action spectra, n =4) and in the absence of retinal (565 nm, n =6). Amplitudes of Arch3 were recorded at the highest transmission of 0.080–0.110 mW mm −2 (at maximal transmission between 500 and 565 nm). Displayed are means±s.e.m. ( d ) Action spectra of HEK cells transfected with Arch3-EGFP in presence of ATR ( n =3), analogue VII ( n =7) or analogue VIII ( n =8). DMAR and analogue IX were also tested but did not enable photocurrents. Displayed are stationary currents following photostimulation at a holding potential of 0 mV (equal photon flux for each wavelength of 2.81 × 10 14 photons s −1 mm −2 ). In ( a ) and ( b ) n values refer to animals, in ( c ) and ( d ) n values refer to cells. Full size image For Mac, ATR mediated a maximal increase in body length at 540 nm (4.5±0.6%; n =7; Fig. 5b , Supplementary Fig. 9b ). Similar action spectra were obtained with naphthyl- and thiophene-retinal, also peaking at 540 nm, but the operational cellular sensitivities with these chromophores were reduced compared with ATR (2.9±0.6%, n =11; 2.2±0.5%, n =7, respectively). DMAR was also less efficient (540 nm; 3.1±0.3%; n =10), especially in the blue, whereas it nearly reached ATR efficiency close to 600 nm. Trimethoxy-retinal (IX) showed no activity in Mac. In a parallel set of experiments, HEK cells transfected with Arch3 were tested in combination with the same retinal analogues. Generally, Arch3 produced rather small photocurrents in this expression system compared with ChR2 at the respective action spectra peaks ( Fig. 5c ; 0.150 mW mm −2 ). This may be explained by a more efficient targeting of ChR2 to the plasma membrane in the stable cell line (compared with transiently transfected Arch3-expressing HEK cells) and by the fact that passive ion transfer through channels is generally larger than vectorial transport through pumps (one ion per absorbed photon). Similar to cells expressing ChR2 ( Fig. 3f ), HEK cells in the absence of retinal showed minor currents (7±2 pA; n =6; Fig. 5c ), although measured in retinoid-deprived culture medium without FCS (fetal calf serum). Similar to C. elegans , DMAR and analogue IX did not enable any currents (both 0±0 pA; n =4). The largest effects were obtained in the presence of analogue VIII (42±13 pA; n =5), while analogue VII (30±7 pA; n =4) showed the same effectiveness as ATR (34±5 pA; n =14). Both analogues that showed functionality featured a large blue shift in the action spectrum (30 and 60 nm shifts for analogues VIII and VII, respectively), which was comparable to the shifts observed for Arch3 in C. elegans BWMs ( Fig. 5d ). We could not compile an analogous data set for Mac, as this protein showed poor plasma membrane targeting. We characterized eight synthetic retinal analogues for their potential to reconstitute and modify function in several rhodopsin-based optogenetic tools, in vivo , compared with the natural chromophore ATR. Our results (summarized in Table 1 ) show, first, that artificial analogues of ATR can be successfully used for colour tuning of rhodopsins; second that the colour shifts varied between different rhodopsins; and third that analogues may also affect photocycle kinetics. Table 1 Summary of key results presented in this study. Full size table DMAR promoted ChR2-evoked behavioural effects in C. elegans with a significantly red-shifted action spectrum compared with ATR (maxima for ATR at 480 nm and DMAR at 500–568 nm). The light sensitivity of cells was increased, particularly at the red edge of the spectrum (12 times compared with ATR). An even bigger sensitivity gain and a 40-nm spectral red-shift was obtained for the ChR2(H134R/T159C)/DMAR combination. At all wavelengths tested, strong body contractions could be achieved even at 0.004 mW mm − 2 , 50- to 100-fold less light than that used to achieve similar effects with ChR2(H134R)/ATR. This was due to the improved expression of ChR2(H134R/T159C) (ref. 20 ) and extended open-state life time, resulting in more charge transfer per photocycle. Thus, DMAR provides an alternative to achieving higher operational light sensitivity of the cells at red-shifted wavelengths, at still comparably fast on and off switching of the channel. Provided that DMAR can be supplied to organotypic cultures or animals in amounts sufficient to replace the endogenously present ATR, DMAR may facilitate photostimulation deep within tissue, with red light that is less prone to scattering. In C. elegans , the increased operational light sensitivity of BWMs combined with the red-shifted spectrum furthermore helps to avoid photophobic responses that are evoked during prolonged activation with intense blue light [63] and which may interfere with specific, ChR2-evoked behavioural effects in neuronal circuit studies. One important model system in the neurosciences, Drosophila , has been particularly ‘resistant’ to the use of wild-type ChR2 in the central nervous system of adult flies. Recent work using the red-shifted variants ReaChR [32] or Chrimson [33] could overcome this limitation to some degree, possibly due to the higher operational cellular sensitivity, red-shifted absorption and ease of tissue penetration of red light. We show that already existing ChR2 Drosophila lines can be rendered more sensitive to red light using DMAR. However, the problem of most ChR variants being rather inefficient in the central nervous system of adult Drosophila could not be overcome. A recent ChR variant (ChR-XXL) with good expression and extremely long photocycle provides a very promising solution for this problem [57] . The retinal analogues V, VII, VIII and IX were also functional and caused a modest blue-shift in the ChR2 action spectrum (436 nm; Table 1 ). These shifts are likely not distinct enough to allow a meaningful combination with GECIs for Ca 2+ imaging without the cross-activation of ChR2 ( Supplementary Fig. 10 ). On the other hand, analogues III, IV and VI did not mediate relevant muscle contractions, possibly because these chromophores only weakly bind to and weakly stabilize ChR for trafficking. Significant deceleration of channel kinetics was observed for analogues VIII and IX, with the latter mediating particularly strong currents in HEK cells. Possible reasons for altered channel kinetics are that the retinal analogues are embedded slightly twisted in the apoprotein and/or that they interact differently with side chains, thus changing the transition barriers between photocycle intermediates; this needs to be analysed by spectroscopy on isolated and reconstituted protein. Determining how retinal analogues influence kinetic and spectral properties may permit rational design of further synthetic analogues. Interestingly, retinal analogues had different effects on ChR2 (ATR: maximum 465 nm) compared with the red-shifted hyperpolarizer Arch3 (ATR: maximum 560 nm) in HEK cells: Analogues that were functional in ChR2 did not support Arch3 function (II, IX). A comparison of currently available crystal structures of C1C2 (a chimera between ChR1 and ChR2) and Arch2 indicates that the spacious analogue IX (covalently docked) may be less stabilized in Arch, and that steric clashes can be observed which could hinder binding ( Supplementary Fig. 11 ). Our findings suggest that slight modifications of the chromophore often lead to a slowdown of photocycle kinetics. This can be deteriorating for ion pumps that depend on high turnover, but not for channels that rather exhibit longer open-state lifetimes. Furthermore, the opsin shift (absorption maximum of unbound retinal relative to the rhodopsin action spectrum maximum) in the case of Arch3 by analogues VII (360→500 nm) and VIII (400→530 nm) was less pronounced than for ATR (380→560 nm). The opsin shift might be limited in red-shifted optogenetic tools where it is in part caused by polar amino acids in the binding pocket [64] . Most retinal analogues we tested were already more polar near the ring than ATR. Thus, the polar characteristics of the analogues may not sum up with effects by more polar amino acids in ‘red-shifted’ rhodopsins that prevent DMAR binding in the case of C1V1 (ref. 20 ). The non-functionality of certain retinals in some of the opsins, but not in others, opens up a new avenue for orthogonal retinal/rhodopsin pairs where the respective retinals interact specifically and exclusively only with one of the rhodopsins. As a novel strategy, it is conceivable to simultaneously use two (or more) rhodopsins in the same animal that are each supplemented with a specific retinal analogue. This might allow for the combined use of different rhodopsins with specifically altered properties. Replacing ATR in a tissue or in an organism by a synthetic analogue requires the procurement and exogenous application of the chromophore. This is not a significant limitation of the approach if the retinal analogue is able to out-compete endogenous ATR for binding to the optogenetic tool. It is particularly straightforward in model systems such as C. elegans , which need to be supplemented with the chromophore anyway. Optogenetic tools with modified action spectra may promote the possibility of stimulating cells with ChR and simultaneously imaging Ca 2+ . This is precluded for most GECIs by the broad action spectra of available rhodopsins ( Supplementary Fig. 10 ). Only the novel Ca 2+ sensor RCaMP has so far been applied without the unintended co-activation of ChR2 (refs 1 , 18 , 38 , 65 , 66 ). Testing more retinal analogues may allow the identification of additional combinations of optical sensors and rhodopsin actuators. The analogues we characterized unfortunately do not permit enough spectral shift to achieve this goal. In this work, we carried out a survey of entirely artificial, synthetic retinal analogues directly in mammalian cells and in vivo in C. elegans and Drosophila larvae. Our results illustrate that matching ChR variants and other rhodopsins with synthetic retinal analogues can generate optogenetic tools with modified characteristics with respect to absorption spectra and kinetics. Thus, the study opens the door to further optimization by combining rhodopsin-based optogenetic tools with (synthetic) retinal analogues. This may help to improve the performance of such tools, with the potential for developing additional combinations that might offer the particular characteristics required for a specific application. Synthesis of retinal analogues The synthesis of some of the retinal analogues has been described previously [46] . Details of the synthesis of compounds II–IX, as well as 1 H NMR, 13 C NMR and HMRS data, can be found in Supplementary Methods . Absorption spectra were measured in isopropanol (0.02 mM) with BioSpectrometer Basic (Eppendorf, Germany). C. elegans strains C. elegans strains were cultivated in the dark at 20 °C on nematode growth medium (NGM) plates in the presence of the E. coli strain OP50-1 (ref. 67 ). The following transgenic strains were used: ZX299: lin-15(n765ts−); zxEx22[pmyo-3::ChR2(H134R)::YFP; lin-15+] (ref. 50 ); ZX980: wild type; zxEx516[pmyo-3::C1V1(E122T; E162T)::YFP; pmyo-2::mCherry]; ZX1166: wild type; zxEx536[pmyo-3::ChR2(T159C)::YFP; pmyo-2::mCherry]; ZX1167: wild type; zxEx537[pmyo-3::ChR2(H134R; T159C)::YFP; pmyo-2::mCherry] (all from ref. 20 ); ZX1483: lin-15(n765ts); zxEx820[pmyo-3::Arch3::2xmyc-tag; lin15(+)]; ZX1484: lin-15(n765ts); zxEx821[pmyo-3::Mac::2xmyc-tag; lin15(+)] C. elegans behavioural assays C. elegans strains were kept under light-excluding conditions on standard NGM plates (5.5 cm diameter; 8 ml NGM). Per plate, 300 μl of OP50-1 culture containing either 250 μM (ChR2) or 100 μM (Arch3, Mac) of ATR or retinal analogue (diluted in ethanol) were spread and allowed to dry, before worms were added. The day before the experiment, transgenic L4 larvae were selected for muscle fluorescence and light reactivity under a Leica MZ16F dissection scope and transferred to fresh chromophore plates. Resulting young adults were again selected and transferred to NGM plates with OP50-1 bacteria provided with either ATR or the respective retinal analogue at least 2 h before the experiment. For measurements of contractions and elongations [20] , [67] , worms were individually placed on plain NGM plates and assayed on an Axiovert 200 microscope with × 10 magnification (Zeiss, Germany). For colour illumination, the light of a 100-W mercury arc lamp was channelled through a beamsplitter (F38–651, AHF Analysentechnik, Tübingen, Germany) and excitation BP filters of 400±10 nm, 436±10 nm, 480±10 nm, 520±10 nm, 540±10 nm, 568±10 nm, 580±10 nm or 600±10 nm (Edmund Optics, Karlsruhe, Germany). Alternatively a rhodamine (540±35 nm) or a Cy5 filter (620±30 nm) was used (AHF Analysentechnik, Tübingen, Germany). Intensities were individually adjusted using the lamp intensity control panel and neutral density filters (Zeiss, Germany), as defined by the S120 UV Sensor with PM 100 power meter (Thorlabs, Dachau, Germany). In consecutive recordings of initially forward-moving animals, using a CMOS camera (DCC1545M, Thorlabs, Dachau, Germany), HBO illumination on- and offset were defined by a computer-controlled shutter (Sutter Instruments, USA). Only those movies were taken into account in which the animals did not display backward locomotion at least until the end of the light stimulus. All frames were extracted for body length using a custom written LabView script [11] , and the percentage length relative to the body size of each worm before illumination was calculated and averaged [20] . Displayed are means±s.e.m. Electrophysiology in C. elegans C. elegans strains were kept under light-excluding conditions on high-growth medium plates (9 cm diameter; 25 ml high-growth medium). Per plate, 650 μl of OP50-1 culture containing ATR or DMAR (250 μM; diluted in ethanol) were spread and allowed to dry before worms were added. Electrophysiological recordings were performed from dissected BWMs [4] . After dissection, cells were treated for 8 s with 0.5 mg ml −1 collagenase (Sigma, Germany) in C. elegans Ringer’s (CRG; 150 mM NaCl, 5 mM KCl, 5 mM CaCl 2 , 1 mM MgCl 2 , 10 mM glucose, 15 mM HEPES (pH 7.35), 340 mOsm) and washed with CRG. Cells were clamped to a holding potential of −60 mV using an EPC10 amplifier with head stage and Patchmaster software (HEKA, Germany). The bath solution was CRG, the pipette solution was 120 mM KCl, 20 mM KOH, 4 mM MgCl 2 , 5 mM TRIS-HCl, pH 7.2, 0.25 mM CaCl 2 , 4 mM ATP, 36 mM sucrose, and 5 mM EGTA, 315 mOsm. Light activation was performed using an LED (light-emitting diode) lamp at a wavelength of 470 nm (KSL-70, Rapp OptoElectronic, Germany) or 525 nm (LumenLED, Prior Scientific Instruments, Germany), and controlled by Patchmaster software (HEKA, Germany). Light intensity applied was 0.2 mW mm −2 using lamp intensity control panel and neutral density filters (Zeiss, Germany) as defined by an S120 UV Sensor with PM 100 power meter (Thorlabs, Dachau, Germany). Only previously unstimulated animals were used for each single experiment. For the analysis, ASCII data files were analysed with Origin software (OriginLab, Northampton, MA, USA). Electrophysiology in HEK cells Serum-free culture of HEK cells . Advanced DMEM (Life Technologies, USA) was used as culture medium without supplementation with FCS to prevent contamination by retinoids from serum. Culture flasks (TPP, Switzerland) were coated with poly- L -lysine (Biochrome, Germany) to maintain adhesion. Coverslips were shortly heated in fire, coated with poly- L -lysine and put into dishes with 2 ml advanced DMEM per dish. Measurements were accomplished using the stable ChR2-YFP cell line [68] and HEK-293 cells (DSMZ no. ACC-305). After 1 week, the expression of ChR2 was induced by the addition of tetracycline (to a final concentration of 2 μM), whereas the expression of Arch3-EGFP was achieved by transient transfection of HEK-293 cells with FuGENE HD (Promega, Madison, WI, USA). Stock solutions of retinal analogues were stored in the dark (1 mM, dissolved in isopropyl alcohol). The respective retinal analogues were added to the dishes at a final concentration of 1 μM directly after induction/transfection. Recording of photocurrents . Photocurrents were determined by the whole-cell patch-clamp technique 24–30 h after induction/transfection. A Polychrome V (TILL Photonics, Germany) was used as the light source and controlled via TillVision software (TILL Photonics, Germany) and a VS25 shutter (Vincent Associates Uniblitz, USA). Action spectra were recorded at light intensities that were directly adjusted to an equal number of photons (2.81 × 10 14 photons s −1 mm −2 ) for all wavelengths using a motorized filter wheel (NSND-3, Newport, Irvine, CA, USA). For comparison with other experiments, illumination with blue light of 470 nm corresponded to a light intensity of 0.119 mW mm −2 . To establish action spectra for ChR2, we conducted 10-ms illuminations using an additional 10% grey filter for each wavelength (2.81 × 10 13 photons s −1 mm −2 ). At a holding potential of −60 mV, the transient peak current was analysed to exclude an activation of photointermediates. For the action spectra of Arch3, we conducted 300 ms illuminations for each wavelength. Because for this pump a transient peak was not or only barely visible, the stationary current at a holding potential of 0 mV was analysed. To measure current amplitudes, we conducted 300-ms illuminations and analysed stationary currents with excitation at 465±7 nm (ChR2; all retinal analogues), 565±7 nm (Arch3; ATR), 530±7 nm (Arch3; VIII) or 500±7 nm (Arch3; VII). Further details are given in the respective figure legends. The external bath solution contained [mM]: 140 NaCl, 1 CaCl 2 , 1 KCl, 1 MgCl 2 and 10 HEPES (pH 7.2 adjusted with NMG), whereas the intracellular pipette solution contained [mM]: 110 NaCl, 10 EGTA, 5 KCl, 1 CaCl 2 , 1 MgCl 2 and 10 HEPES (pH 7.2 adjusted with NMG). Behavioural assays on larval Drosophila Third instar larvae, 5–6 days of age after egg-laying, were used. Larvae expressing UAS:ChR2(H134R) (ref. 59 ) under the control of the Actin-Gal4 driver were raised at 25 °C on standard medium containing either 125 μM ATR (Sigma, Heidelberg, Germany) or DMAR, both dissolved in ethanol (10 μl of solution in 10 ml food). As a control, animals raised on medium containing ethanol only were used. To observe light-induced muscle contractions, individual larvae were placed on a coverslip and illuminated from below with a custom-built illuminator containing high-power LEDs (Huey Jann, electronics industry Co., Wu-Chi Town Taichung Shien, Taiwan) of wavelength 465, 520, 590 and 625 nm, respectively. Larvae were observed using a stereomicroscope (Discovery.V8, Zeiss, Oberkochen, Germany) equipped with a AxioCam MRm camera. Contractions of the whole larvae in response to light stimulation were observed under dim white light illumination (~0.0002, mW mm − 2 ). Muscle contractions induced by monochromatic light were measured for each wavelength at ~0.01, ~0.02, ~0.07 and ~0.1 mW mm − 2 . Light intensities were controlled with a custom-built power supply and calibrated using a photometer (Lasercheck, Coherent, Santa Clara, CA, USA). Structure visualization For structure visualizations, PyMOL (Schrödinger, Germany), Molecular Operating Environment 2013.0802 (CCG, Canada) and GOLD 5.2 (CCDC, UK) were used. The molecular structure files for the proteins (PDB IDs: 3UG9 and 1VGO) and the ligand (analogue IX) were prepared in MOE. To predict the best possible binding modes of the ligand, docking was carried out using GOLD. The binding site was centered at the lysine residue of the protein involved in Schiff base formation with the chromophore and all surrounding atoms of the active-site within 20 Å were selected. The covalent bond was specified between the ε–N of the lysine of the protein and the ligand. The best protein–ligand docked binding mode was chosen based on the CHEMPLP score. The default docking parameters were used. Statistics Sample size was chosen so that the statistical significance could be achieved within the measurement accuracy of the respective experiment. All of the samples recorded were included in data analysis. Statistical analysis was carried out with Microsoft Excel, Prism (GraphPad, USA) or Origin (OriginLab, USA). Significance is given as P value after two-tailed Student’s t -test, one-way analysis of variance with Bonferroni’s or Fisher’s post hoc test, two-way analysis of variance or χ 2 -test: NS not significant, * P <0.05; ** P <0.01; *** P <0.001. For the elongation experiments in C. elegans , we compared data in the time window 4.5–6.5 s of retinal analogues to controls that were raised in the absence of any chromophore. Time constants were obtained by non-linear fitting for monoexponential decay of body length or inward current changes using Origin (OriginLab). How to cite this article: AzimiHashemi, N. et al . Synthetic retinal analogues modify the spectral and kinetic characteristics of microbial rhodopsin optogenetic tools. Nat. Commun. 5:5810 doi: 10.1038/ncomms6810 (2014).